Polaron hopping mediated by nuclear tunnelling in semiconducting polymers at high carrier density The transition rate for a single hop of a charge carrier in a semiconducting polymer is assumed to be thermally activated. As the temperature approaches absolute zero, the predicted conductivity becomes infinitesimal in contrast to the measured finite conductivity. Here we present a uniform description of charge transport in semiconducting polymers, including the existence of absolute-zero ground-state oscillations that allow nuclear tunnelling through classical barriers. The resulting expression for the macroscopic current shows a power-law dependence on both temperature and voltage. To suppress the omnipresent disorder, the predictions are experimentally verified in semiconducting polymers at high carrier density using chemically doped in-plane diodes and ferroelectric field-effect transistors. The renormalized current-voltage characteristics of various polymers and devices at all temperatures collapse on a single universal curve, thereby demonstrating the relevance of nuclear tunnelling for organic electronic devices. Basic electronic components such as transistors, light-emitting diodes and solar cells made from conjugated polymers are currently investigated for a wide range of applications such as displays, smart labels and photovoltaics. The semiconducting properties in conjugated polymers stem from the covalent interactions between the monomers on the backbone of the π-conjugated polymer [1] . Although polymer chains provide a conjugated path for charge transport, real devices offer only limited charge mobility due to the presence of disorder, which disrupts the π-conjugation, and due to polarization of the surrounding medium, which augments the effective mass of the charge carriers. As a consequence, charges are localized over small segments, yielding spatially and energetically distributed transport sites. Electrical conduction occurs by hopping, which is thermally assisted tunnelling of charge carriers between localized sites. In the semi-classical approach, the transition rate for a single hopping event is given by: where the barrier E A arises due to disorder between sites and due to nuclear polarization. Insight into the transport physics of these dissipative systems is provided by models that link the microscopic parameters found in the transition rate to macroscopic currents as measured in experiments. In the semi-classical approaches of Miller–Abrahams (M–A) and Marcus, to be discussed below, it is assumed that the transition rate is thermally activated and expected to vanish when the temperature approaches absolute zero. Numerous experiments, however, have shown that the conductivity at low temperatures is finite [2] , [3] , [4] , [5] , [6] . Therefore, the semi-classical approaches breakdown at low temperatures. Reported explanations artificially assume two transport regimes, a thermally activated one at high temperature and an activation-less transport mechanism at low temperatures [4] , [5] , [6] . A unified description of charge transport through disordered π-conjugated polymers for a wide temperature and voltage range is therefore lacking. Here we show that the semi-classical description breaks down, because even at absolute zero, the quantum mechanical zero-point energy of the system exists. The ground-state oscillations that drive the nuclear tunnelling then become important. We present a uniform description of charge transport in highly doped semiconducting polymers by quantum mechanical treatment of the system. We derive an expression for the macroscopic current based on the transfer rate for nuclear tunnelling. The current shows a power-law dependence on both temperature and voltage. The renormalized current-voltage characteristics of various polymers and devices at all temperatures collapse on a single universal curve. The universality of the curve proves that the charge transport in all polymers is similar and driven by nuclear tunnelling. Semi-classical description of hopping An expression for the hopping transition rate is given in the seminal paper of M–A in 1960 ( [7] ). The M–A hopping rate, with the simplifications as introduced by Ambegaokar [8] , has been the basis for models describing charge transport in disordered semiconductors [9] . In this formalism, the activation energy E A represents the energy difference between the initial and final state, whereas the prefactor k 0 depends exponentially on the distance between the sites, as shown in Fig. 1a . For hops downhill in energy, the hopping rate is just given by k 0 . 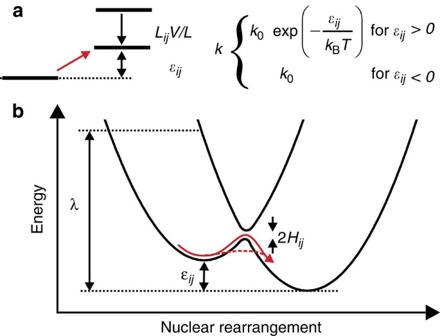Figure 1: The hopping mechanisms. (a) Schematic representation of the M–A hopping process. (b) Schematic representation of electron transfer in a biased double quantum well.λis the reorganization energy,εijis the difference in minimum of the potential energy wells andHijis the tunnel splitting. The semi-classical Marcus hopping path and the nuclear tunnelling mechanism are indicated by solid-red and dashed-red arrows, respectively. A macroscopic current results when a voltage V is applied over a semiconductor with length L as the energy difference is lowered by the electric field: Figure 1: The hopping mechanisms. ( a ) Schematic representation of the M–A hopping process. ( b ) Schematic representation of electron transfer in a biased double quantum well. λ is the reorganization energy, ε ij is the difference in minimum of the potential energy wells and H ij is the tunnel splitting. The semi-classical Marcus hopping path and the nuclear tunnelling mechanism are indicated by solid-red and dashed-red arrows, respectively. Full size image where L ij is the distance between the initial and final state, that is, the hopping length. Models for the macroscopic conductivity follow from path optimization of hopping distance and difference in energy levels involved [10] . The M–A formalism is applicable to systems where the transport is dominated by energetic disorder. This is typically the case in semiconducting polymers at low charge carrier density. In this regime, the concept of the transport energy has been introduced to account for the critical influence of the shape of the density of states (DOS) on the macroscopic currents. The strong dependence on the DOS renders the derivation of a universal description difficult as tail states in the DOS are often a consequence of chemical impurities or grain boundaries and do not necessarily represent the intrinsic transport characteristics of the polymer. In systems where the activation barrier arises either owing to dynamic disorder or due to the relaxation of local nuclear configurations (polarization), the static energetic disorder picture of the M–A formalism fails. Here we focus on the effect of the local nuclear configurations as taken into account in the Marcus electron transfer theory. The polarization effects are included in the transition rate that depends on the electronic coupling between the initial and final state and the reorganization energy λ , which is twice the polaron-binding energy, as schematically indicated in Fig. 1b ( [11] ). There are two potential energy wells where the polaronic charge carrier can be localized. In an applied electric field of V/L , the two minima of the potential energy wells, , differ again by: The shape of the two parabolas is determined by the reorganization energy λ . Assuming that the tunnel-splitting H ij is small, the activation energy E A , which is equal to the barrier for hopping, is then: The macroscopic current can be derived by assuming that the polarization-induced barriers prevail and that disorder can be neglected as a consequence of high charge carrier density. In this approximation, it has been calculated [12] and experimentally verified [13] , [14] that as the carrier density increases, the charge transport is less dependent on subtleties of the DOS tail, and that the transport occurs closer to the Fermi level. As a consequence, all the hopping steps that the polaron carriers have to take to get from one electrode to the other are identical, and the current can be derived by considering the difference between backward and forward hopping. In the case that λ> , the current reads as: In both the M–A and the Marcus approach, the transition rates are thermally activated and vanish when the temperature approaches absolute zero. Numerous experiments, however, have shown that the conductivity at low temperatures is finite [2] , [3] , [4] , [5] , [6] . The breakdown of the semi-classical approaches at low temperatures is due to quantum mechanical zero-point energy of the system. The ground-state oscillations drive the nuclear tunnelling as the temperature approaches absolute zero. Here we present a uniform description of charge transport in semiconducting polymers, including the existence of absolute-zero ground-state oscillations that allow nuclear tunnelling through classical barriers. Nuclear tunnelling In general, it is assumed that hopping is by tunnelling in an asymmetrically biased double quantum well. The charge transfer is driven by the coupling to classical nuclear vibrations that constitute a so-called heat bath. In the classical limit, however, these fluctuations vanish with decreasing temperature. Hence, the semi-classical models predict that the macroscopic current vanishes if the temperature approaches absolute zero. However, even at absolute-zero temperature, the system possesses a quantum mechanical ‘zero-point energy’. The ground-state oscillations drive the tunnelling of the carrier between the initial and final state. Because the shape of the potential originates from the coupling of the electronic charge to its nuclear environment, this tunnelling process is known as nuclear tunnelling to distinguish it from the semi-classical Marcus theory. As a consequence, the tunnelling rate does not decrease to zero at low temperatures, but the charge transfer rate then becomes temperature independent. The importance of nuclear tunnelling for non-adiabatic charge transfer reactions or small polaron hopping was early predicted by theory following the works of Jortner [15] , Emin [16] and Gorhambergeron [17] . Starting from perturbation theory, rate expressions were derived in which single acoustic or optical phonon modes drive the charge transfer and which were treated quantum mechanically. Especially at low temperatures where nuclear tunnelling is pronounced, details of the spectral density of the phonon bath become important, and the influence of phonon freeze out on transport has been discussed. [8] , [10] However, multi-phonon models based on a detailed structure of the coupled phonon spectra can only be solved by extensive numerical calculations to derive the macroscopic current. Examples can be found for small-molecule organic semiconductors in a band-like transport regime [18] , [19] , [20] . For the purely dissipative case, as represented by semiconducting polymers, a compact rate expression that includes nuclear tunnelling driven by the coupling to a full phonon bath has been derived in the seminal papers of Weiss et al . [21] , [22] and Dorsey et al . [23] based on the Spin-Boson Model. For the general case of an Ohmic spectral density with an upper cut-off to describe the coupling between the charge and the nuclear bath, the transfer rate is given in the non-adiabatic limit as: where H ij is the electronic coupling between initial and final state, ε ij is the energy difference between donor and acceptor states, α′ is the Kondo parameter describing the coupling strength between charge and bath, ω c is the characteristic frequency of the bath and Γ denotes the complex gamma function. The classical reorganization energy associated with the bath is ( [24] ). We note that in the high temperature limit ( ), the formalism leading to expression (6) reduces to the semi-classical Marcus electron transfer theory [11] , [24] . We remark that nuclear tunnelling is only a metaphor for a proper quantum mechanical description of the heat bath. The main reason why the quantum mechanical description is so important in semiconducting polymers is that the characteristic frequency of the heat bath is rather high. Marcus theory works well for redox reactions in water and charge transfer in proteins. In these polar environments, low-frequency rotational vibrations and other solvent modes are treated classically. In a non-polar semiconducting polymer, the charge moves mainly due to changes in bond length. The relevant stretching vibrations are at high frequency, and still at room temperature, most of the states are in the vibrational ground state, which is completely different from a classical oscillator. To calculate the macroscopic current using the left-hand side of equation (5), assuming identical hopping steps, the applied potential V again enters via , where γ − 1 is equal to the number of hopping events needed for charge carriers to traverse the distance between the electrodes, L . Assuming and by replacing , the current is given by: As a result, with the rate expression given by Weiss et al ., a single analytic expression can be derived linking the macroscopic current with parameters derived from microscopic theories. This I(V, T) relation shows a power-law dependence on temperature in the low-voltage Ohmic regime, given by: Additionally, equation (7) describes a second high-voltage regime where the current is temperature independent and follows a power-law as a function of bias: Intuitively, the crossover between the two transport regimes is expected at the voltage where the carrier’s potential electrical energy for a single hop eV hop is equal to the carrier’s thermal energy k B T . Depending on eV hop / k B T , the driving force for a single hop changes. When eV hop / k B T <<1, the current is Ohmic with power-law dependence on temperature, and when eV hop / k B T >> 1, the current is superlinear in electric field and almost temperature independent. We note that other physical models yield a similar functional dependence for current as a function of voltage and temperature, for example, variable range hopping [25] , Luttinger Liquid [2] , [26] and Coulomb blockade [3] , [27] . All these models are mutually exclusive and inconsistent with each other. For instance, Luttinger Liquid is valid for a system free of localization, whereas variable range hopping holds for systems with localized states. Design of experiment To experimentally verify nuclear tunnelling, the role of energetic disorder [28] must be suppressed, because the derivation of equation (7) is based on the assumption that the transport is characterized by a sequence of equal hopping steps, whereas the presence of energetic disorder mandates otherwise. To eliminate the effects of the energetic disorder, we measure transport at high charge carrier densities. When the DOS is filled up with carriers, the density of available states near the Fermi level is large. The charge carriers then hop between sites with a narrow energetic spreading, that is, ‘nearly’ energetically similar states. Therefore, energetic disorder is suppressed and disentangled from the intrinsic hopping mechanism. To secure the assumption behind equation (7), we used ferroelectric field-effect transistors (FeFET), where the high carrier density is achieved by the ferroelectric polarization of the gate dielectric [29] , and we used in-plane diodes with highly chemically doped polymers [30] . High carrier densities enable conductivity measurements at very low temperature and at a very low voltage. Hence, the voltage could be varied over five orders of magnitude over a temperature from 10 to 300 K. We note that the maximum volume density in the FeFET amounts typically to one charge carrier per 30 monomeric units. As a result, correlation effects between charge carriers can be disregarded, as confirmed by Paulsen et al . [31] Experiment Among the studied materials, we used regio-regular poly(3-hexylethiophene) (rr-P3HT), which is extensively studied in solar cells, poly[2-methoxy-5(3′,7′-dimethloctyloxy)-1,4-phenylene vinylene] (OC 1 C 10 -PPV), the workhorse for polymer light-emitting diodes and poly[bis(4-phenyl)(2,4,6-trimethylphenyl)amine] (PTAA), which has been extensively investigated in thin-film transistors. The microstructure of the films ranged from semi-crystalline to amorphous. The FeFET layout and the chemical structures of the polymers used are presented in Fig. 2a . The bottom-contact/top-gate FeFET were made using the random copolymer poly(vinylidene fluoride-trifluoroethylene) (P(VDF-TrFE) (65–35%)) as ferroelectric gate dielectric and rr-P3HT or PTAA as semiconductor. For transport measurements using in-plane diodes, we used rr-P3HT and OC 1 C 10 -PPV as semiconductor, both heavily doped by vapourized trichloro-1H,1H,2H,2H-perfluorooctylsilane (TCPFOS). 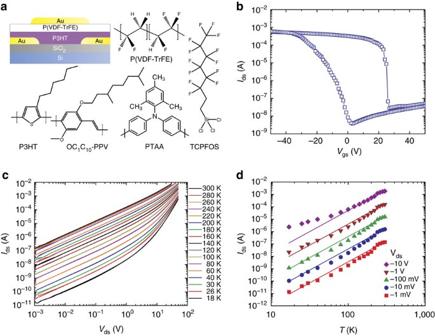Figure 2: Electrical characterization of rr-P3HT FeFET. (a) Layout of a top-gate FeFET, and chemical structures of the compounds used. (b) Typical transfer characteristics of a rr-P3HT FeFET. The channel length and width are 10 and 10,000 μm, respectively. (c) Corresponding output characteristics of the rr-P3HT FeFET at zero gate bias as a function of temperature. (d) Source-drain current at zero gate bias as a function of temperature for various source-drain biases. Figure 2: Electrical characterization of rr-P3HT FeFET. ( a ) Layout of a top-gate FeFET, and chemical structures of the compounds used. ( b ) Typical transfer characteristics of a rr-P3HT FeFET. The channel length and width are 10 and 10,000 μm, respectively. ( c ) Corresponding output characteristics of the rr-P3HT FeFET at zero gate bias as a function of temperature. ( d ) Source-drain current at zero gate bias as a function of temperature for various source-drain biases. Full size image Electrical characterization of FeFETs A typical transfer curve of a rr-P3HT top-gate FeFET is presented in Fig. 2b . Comparable data have been obtained for PTAA FeFETs. The rr-P3HT FeFET switches between a high/low conductance on/off-state at gate voltages of −/+25 V, which corresponds to the coercive field of the ferroelectric gate. Because rr-P3HT is a p-type semiconductor, the accumulated holes at negative gate bias compensate for the ferroelectric polarization, and the current is enhanced. At positive gate bias, rr-P3HT is depleted from holes, and the FeFET therefore switches from a polarized on-state to a depolarized off-state. Conductance switching only requires polarization of P(VDF-TrFE) at the source electrode. Polarization at the drain is irrelevant and does not impede charge extraction [32] . The high conductance on-state originates from the large surface-charge density induced in the semiconductor channel by the ferroelectric polarization of P(VDF-TrFE) [33] . The induced charge density, ρ , was determined by comparing the current response of non-ferroelectric and ferroelectric transistors, as previously proposed [34] . The induced amount of charge was equal to 20 mC m −2 at zero gate voltage, and shifts the Fermi level into the conduction band of the polymeric semiconductor. The high charge density value allows measurement of the current at drain biases as low as 1 mV. The FeFET was programmed in the high conductance on-state and the output characteristics ( I ds versus V ds ) were measured at zero gate bias. The drain voltage was swept from 1 mV to 100 V and back while the source electrode was grounded. The output curves at temperatures between 300 and 18 K are presented on a double logarithmic scale in Fig. 2c . We note that the current is still larger than the leakage current at temperatures as low as 18 K and at drain biases of 1 mV. Furthermore, the polarization of the P(VDF-TrFE) gate dielectric remained unchanged during the measurements and hysteresis in the output characteristics at all temperatures was negligible. The transport at high temperature is Ohmic, and linear in bias, at all voltages, in accordance with equation (8). The current decreases with decreasing temperature, and at low temperature, the output curves become non-linear, as expected from equation (9). The transition voltage from linear to superlinear behaviour decreases with decreasing temperature. In a small temperature range of 300–140 K, the current at low bias can be approximated with an exponential dependence, exhibiting an activation energy of about 80 meV, a value that is comparable to literature data [35] . However, the exponential Arrhenius approximation is an artefact of the limited temperature range. Figure 2d shows that over the complete temperature range, the current follows a power-law dependence on temperature in agreement with equation (8). A good fit to the data is obtained for biases up to 10 V with a value of α of 3.6. Scaling of charge transport To determine the voltage dependence, we partition the temperature dependence according to equation (7) as . Hence, we present the scaled current I ds /T α+1 , as a function of relative energy eV ds / k B T . The scaled current of rr-P3HT FeFETs with different channel lengths are presented as a function of relative energy, eV ds / k B T , in Fig. 3 , using the experimentally determined value for α of 3.6. For each FeFET, all measurements for different voltages and temperatures collapse onto a single curve. At low values of eV ds / k B T , the scaled current increases linearly with relative energy (equation (8)). At high values of eV ds / k B T , the scaled current increases superlinearly (equation (9)). There is a single crossover point for each channel length. Subsequently, the scaled current of each rr-P3HT FeFET was fitted to equation (7) using the experimentally determined value of the parameter α of 3.6. 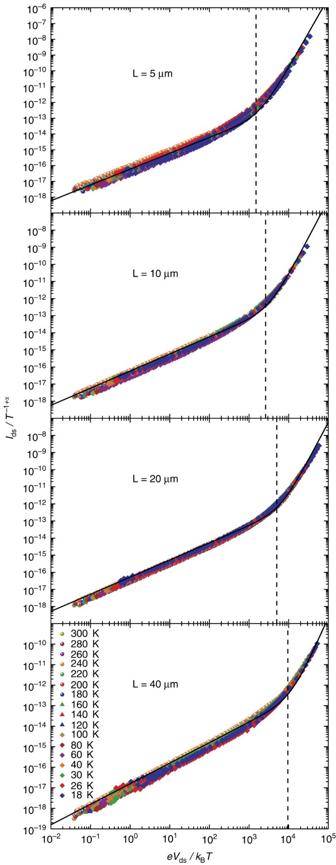Figure 3: Scaling of the current-voltage characteristics of rr-P3HT FeFETs. Scaled source-drain current,Ids/T1+α, as a function of relative energyeVds/kBTof rr-P3HT FeFETs, with different channel length of 5, 10, 20 and 40 μm. The channel width is 10,000 μm. The value ofα=3.6 is determined from the temperature dependence of the current at low bias. The solid lines are fits to equation (7). The dashed vertical lines are a guide to the eye for the position of the crossover in the curves. Figure 3 shows that an excellent fit is obtained for each channel length. Equally good fits were obtained for PTAA FeFET and in-plane diodes of chemically doped rr-P3HT and OC 1 C 10 -PPV. Figure 3: Scaling of the current-voltage characteristics of rr-P3HT FeFETs. Scaled source-drain current, I ds /T 1+α , as a function of relative energy eV ds / k B T of rr-P3HT FeFETs, with different channel length of 5, 10, 20 and 40 μm. The channel width is 10,000 μm. The value of α =3.6 is determined from the temperature dependence of the current at low bias. The solid lines are fits to equation (7). The dashed vertical lines are a guide to the eye for the position of the crossover in the curves. Full size image The parameters α and I 0 do not depend on the length of the channel. The values of I 0 are in the range of 1.2 × 10 − 15 –3.5 × 10 − 15 A/K 1+α . The parameter γ , however, changes with the channel length. The dotted lines in Fig. 3 show the position of the crossover between the linear and the superlinear regime. The position of the crossover, which is uniquely determined by the parameter γ in equation (7), increases with relative energy, eV ds / k B T , as the channel length increases. Within the context of the nuclear tunnelling model, γ −1 is equal to the number of hopping events needed for charge carriers to traverse the channel length. Therefore, a relation between γ − 1 and the channel length, L , is expected. The extracted values of γ − 1 are presented in Fig. 4 as a function of channel length. A linear dependence is obtained. The fit goes through the origin. The zero intercept beautifully shows that, as intuitively expected, in the limit of zero channel length, the number of hops is zero. In our approximation of identical hops, the slope is equal to the number of tunnelling events (or hops) per unit length. A value of 26 nm is then derived for the average distance between the hopping sites, L ij . However, typically hopping distances between 1 and 10 nm have been reported [10] . It should be noted that under the assumption of identical hops, represents the field enhancement of the transport. For disordered organic semiconductors, as considered here, the origin of the field enhancement of the charge carrier mobility is subject of a long-standing discussion. Experimentally, a stretched exponential of the form μ~ exp (γ ) has been found [36] , with γ the field-enhancement factor. To explain this ubiquitous field dependence, Bässler [9] has performed numerical simulations of charge transport in a regular array of hopping sites with a Gaussian distribution of site energies. They were able to reproduce the field dependence only at relatively high electric fields (100–300 MV m −1 ). Experimentally, the stretched exponential was observed even for fields as low as 1 MV m −1 ( [36] , [37] , [38] , [39] , [40] ). As already noted by Gill [36] , the strong field dependence observed at low fields, as also used in our experiments, requires a length scale of at least several molecular spacings. Longer length scales in the transport have been introduced by Gartstein and Conwell [41] by taking into account spatial correlations between the energies of neighbouring sites, which extends the stretched exponential behaviour to lower fields. The stretched exponential form can be correlated to energy correlations associated with charge–dipole interactions, extending over more than 10 hopping sites [42] , similar to the distance obtained from our length scaling. Thus, our assumption of identical hops leads to a universal scaling behaviour, but the characteristic transport length related to the field enhancement in disordered materials should not be interpreted as the neighbouring site distance. 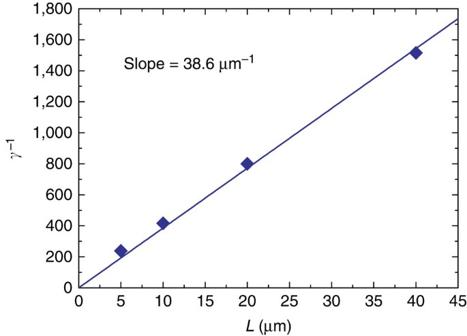Figure 4: Scaling of the number of hops with length. The value of γ−1as a function of channel length,L, for rr-P3HT FeFETs. The solid line is a linear fit yielding a slope of 38.6 μm−1, translating to a characteristic hopping distanceLij, of 26 nm. Figure 4: Scaling of the number of hops with length. The value of γ −1 as a function of channel length, L , for rr-P3HT FeFETs. The solid line is a linear fit yielding a slope of 38.6 μm − 1 , translating to a characteristic hopping distance L ij , of 26 nm. Full size image We note that we also tried to fit the data with the most elaborate model based on variable range hopping [25] . The model, however, failed to describe the experimental data. Furthermore, we tried to fit simpler, one phonon-mode models like the Markus–Jortner model [15] to our data, but only qualitative fits could be obtained. To substantiate the generality of our analysis, we varied the type of polymer in FeFETs, investigated chemically doped polymers in in-plane diodes and interpreted literature data. The charge carrier transport in a FeFET is confined into a thin accumulation layer while in an in-plane diode transport is through the bulk. The polymers in in-plane diodes were chemically doped. All devices showed a power-law dependence of the current on both temperature and voltage. The scaled current shows a crossover. At low values of eV/ k B T , the scaled current increases linearly with relative energy. At high values of eV/ k B T , the scaled current increases superlinearly. The parameter α was obtained for each polymer from the temperature dependence of the current at low bias. The scaled currents of all devices were then fitted to equation (7). In all cases, a perfect fit was obtained. The fit constant I 0 and the average distance between hopping sites, L ij , calculated from the extracted parameter γ are presented in Table 1 . We further included in Table 1 the values extracted from the reinterpretation of literature data for vertical diodes of poly(3,4-ethylenedioxythiophene) poly(styrenesulfonate) (PEDOT:PSS) [3] and poly(2,5-bis(3-tetradecyllthiophen-2-yl)thieno[3,2-b]thiophene) (pBTTT) field-effect transistors [2] . To discriminate between standard Marcus hopping and nuclear tunnelling in undoped polymers, as used for instance in light-emitting diodes and solar cells, electric fields in excess of a few 100 MV m −1 would be required. Experimentally, this field range is at present difficult to access because of the dielectric breakdown of the diodes. Finally, we emphasize that our model is not applicable to high conductive molecular crystals as the non-adiabatic limit is no longer valid. Table 1 Extracted parameters for various polymers Full size table To show that the charge transport mechanism is similar in all the polymers, we renormalize the I (V , T) characteristics according to equation (7). We renormalize data on the x axis to the dimensionless parameter eV hop / k B T , with V hop =γV , representing the applied bias divided by the number of hops. Furthermore, we renormalize the y axis to I / I 0 T 1 +α . 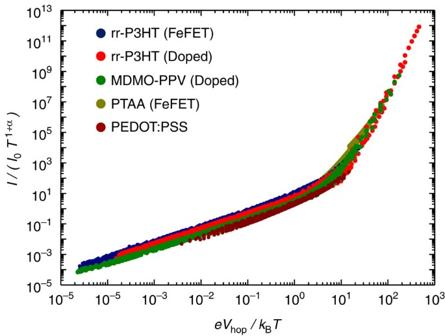Figure 5: Generality of the electrical transport in various semiconducting polymers due to nuclear tunnelling. The scaled current,Ids/I0Tα+1, as a function ofeVhop/kBTon a double logarithmic scale for rr-P3HT and PTAA FeFETs, chemically doped rr-P3HT and OC1OC10-PPV in-plane diodes, and a PEDOT:PSS vertical diode. Each colour represents a set of measurements conducted on devices with different length at 17 different temperatures ranging from 10 to 300 K. Figure 5 shows in a single plot the renormalized data of all the polymers and devices and temperatures. We included PEDOT:PSS in Fig. 5 . The pBTTT data follows the same trend; the extracted values are presented in Table 1 . Figure 5: Generality of the electrical transport in various semiconducting polymers due to nuclear tunnelling. The scaled current, I ds /I 0 T α+1 , as a function of eV hop / k B T on a double logarithmic scale for rr-P3HT and PTAA FeFETs, chemically doped rr-P3HT and OC 1 OC 10 -PPV in-plane diodes, and a PEDOT:PSS vertical diode. Each colour represents a set of measurements conducted on devices with different length at 17 different temperatures ranging from 10 to 300 K. Full size image The plot integrates all measurements at temperatures between 10 and 300 K, with a bias swept over five orders of magnitude. As a consequence of equation (7), all data collapse and a universal curve is obtained. The crossover from linear to superlinear transport occurs when eV hop / k B T is in the order of unity, as expected. To the best of our knowledge, here the first experimental demonstration of nuclear tunnelling for charge transport in semiconducting polymers is reported. In conclusion, we have shown that inclusion of nuclear tunnelling in the hopping rate leads to a unified description of the I(V, T) characteristics of semiconducting polymers at high carrier densities. For all polymers investigated, the full I(V, T) showed a power-law dependence on both temperature and voltage. In a single plot, the renormalized data of all the polymers and devices collapse and a universal curve is obtained. The plot integrates all measurements for different electrode distances, at temperatures between 10 and 300 K, with a bias swept over five orders of magnitude. The universal scaling demonstrates that the charge transport mechanism is similar in all the polymers and occurs via polaron hopping driven by nuclear tunnelling. The mechanism is operational in conventional opto-electronic devices such as organic light-emitting diodes and solar cells. However, then the charge carrier density is low, and disorder is not suppressed. As a consequence, charge carriers have to overcome energetic differences between the localized states at the energetic transport level, in addition to the barriers induced by polarization. For a quantitative analysis, the explicit shape of the DOS then has to be taken into account, which is not trivial and beyond the scope of this paper. Materials The random copolymer of P(VDF-TrFE) (65–35%) was purchased from Solvay and used as received. rr-P3HT was purchased from Rieke Metals. We purified rr-P3HT by dissolving in distilled toluene, dedoping with hydrazine and precipitating in methanol. The precipitate was Soxhlet extracted with methanol, n-hexane and CH 2 Cl 2 until the extraction solvent was colourless. The CH 2 Cl 2 fraction was re-precipitated in methanol, collected, dissolved in chloroform and precipitated again in methanol. The collected fraction was dried under vacuum and stored in a glove box under nitrogen. TCPFOS was purchased from Aldrich and used without purification. OC 1 C 10 -PPV was synthesized in our laboratory. Device preparation Using conventional lithography, 150 nm Au source and drain electrodes were defined using 2 nm Ti as an adhesion layer. The contacts were defined on highly doped silicon wafers with 250 nm of thermally grown silicon oxide. For FeFETs, interdigitated electrodes were used with channel lengths between 5 and 40 μm. The channel width was kept constant at 10,000 μm. The current in FeFETs was measured as zero gate bias. Parasitic leakage currents are small, and interdigitated electrodes can be used. For the doped semiconductors in in-plane diodes, a ring geometry was used. The inner electrode is surrounded by a circular outer electrode, minimizing the parasitic currents. The electrode spacing varied between 0.75 and 40 μm while the electrode width was kept constant at 1000 μm. The in-plane diode substrates were treated with hexamethyldisilazane before semiconductor deposition to passivate the SiO 2 surface. Rr-P3HT was dissolved in chloroform with a concentration of 3 mg ml −1 and spin coated onto the substrate at 4,000 r.p.m. OC 1 C 10 -PPV was dissolved in toluene with a concentration of 3–5 mg ml −1 and spin coated onto the substrate at 3,000 r.p.m. The solutions were filtered through 0.2-μm PTFE filters before spin coating. To dope rr-P3HT and OC 1 C 10 -PPV, the in-plane diode substrates were exposed to TCPFOS vapour in a sealed petri dish inside a glove box for several hours. Rr-P3HT was annealed in vacuum at 140 °C before the doping process. To fabricate FeFETs, after deposition of rr-P3HT, a layer of P(VDF-TrFE) was spin coated at 1,000 r.p.m. from methyl ethyl ketone with a concentration of 100 mg ml −1 . We note that methyl ethyl ketone is an orthogonal solvent for rr-P3HT. The stack was then annealed in a vacuum oven (10 − 1 mbar) at 140 °C to enhance the crystallinity of P(VDF-TrFE). To form the staggered gate of the FeFETs, 70 nm layer of silver was evaporated via a shadow mask. The resulting film thicknesses, measured with a Dektak profilometer, were 20–30 nm for rr-P3HT and 600–1500, nm for P(VDF-TrFE). The top surface of the semiconductor film had a RMS roughness of <1 nm, ensuring a smooth interface between the semiconductor and P(VDF-TrFE). All the preparation processes were conducted in a glove box. Electrical measurements For the FeFETs, first, a gate voltage sweep was performed to set the polarization of P(VDF-TrFE). The FeFETs were then programmed into the high conducting on-state. At all the temperatures, I ds −V ds curves were measured at zero gate bias. We note that sweeping the drain bias to voltages above the coercive field did not influence the high conducting on-state of the FeFET. All electrical measurements were conducted in a cryogenic probe station (Janis Research Co.) with a base pressure of 10 − 5 mbar using a Keithley 4200-SCS Semiconductor Characterization System. How to cite this article: Asadi, K. et al . Polaron hopping mediated by nuclear tunnelling in semiconducting polymers at high carrier density. Nat. Commun. 4:1710 doi: 10.1038/ncomms2708 (2013).